An optimized small molecule inhibitor cocktail supports long-term maintenance of human embryonic stem cells A major challenge in stem cell-mediated regenerative medicine is the development of defined culture systems for the maintenance of clinical-grade human embryonic stem (hES) cells. Here, we identify, using a feedback system control scheme, a unique combination of three small molecule inhibitors that enables the maintenance of hES cells on a fibronectin-coated surface through single cell passaging. After 20 passages, the undifferentiated state of the hES cells was confirmed by OCT4, SSEA4 and NANOG expressions, whereas their pluripotent potential and genetic integrity were demonstrated by teratoma formation and normal karyotype, respectively. Our study attests to the power of the feedback system control scheme to quickly pinpoint optimal conditions for desired biological activities, and provides a chemically defined, scalable and single cell passaging culture system for hES cells. Although the derivation and culture of human embryonic stem (hES) cells has been continuously evolving since the first publication over a decade ago [1] , currently used procedures are usually not well defined, may be contaminated by pathogens or xenogens [2] , and/or cannot support single cell passaging [3] . To circumvent these challenges, many laboratories have focused on developing defined conditions for hES cell culture [4] , [5] , [6] , [7] , [8] , [9] . One strategy has been to replace non-human products, that is, animal sera and mouse embryonic fibroblast (MEF) feeder cells, with defined components of human origin [10] , [11] , [12] , [13] , [14] , [15] . Other studies attempted to completely eliminate the need for feeder cells by introducing surface substrates, feeder cell-conditioned medium and various cytokines and growth factors to support the maintenance of hES cell culture [4] , [6] , [9] , [16] , [17] , [18] , [19] , [20] , [21] , [22] . In addition, Watanabe et al . [3] demonstrated that inhibition of Rho-associated kinase (ROCK) by a small molecule Y27632 could overcome the massive cell death associated with hES cell dissociation during routine passage. Nevertheless, these defined formulations cannot meet one or more of the above-discussed criteria (that is, pathogen/xenogen free, fully defined and permissive for single cell culture) and are often inconsistent compared with the traditional hES cell culture supplemented with serum and feeder cells [1] . In this study, we aimed to identify the optimal combination and concentration of multiple small molecules to replace serum and feeders and allow the maintenance of hES cells through single cell passaging. However, signalling pathways associated with hES cell self-renewal are not fully identified [23] , [24] , making the identification of a unique combination of small molecule inhibitors rather difficult. Furthermore, the combination of a number of inhibitors at various dosages can form a massively large test space. To efficiently identify an optimal cocktail of small molecule inhibitors, we used a feedback system control scheme that has been previously used for searching optimal drug combinations for viral infection inhibition [25] and reactivation [26] . Using this scheme, we discovered a unique combination of three small molecule inhibitors, which with supplement of basic fibroblast growth factor (bFGF) supports long-term maintenance of hES cell culture through routine single cell passaging, as evidenced by various pluripotent marker expressions, teratoma formation and normal karyotype. 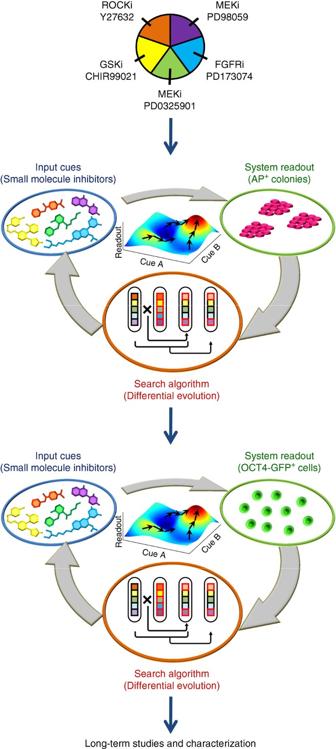Figure 1: A schematic illustration of our experimental design. Through literature search, five small molecule inhibitors targeting key pathways involved in hES cells were selected. Combinations and concentrations of the five inhibitors were optimized using the feedback system control scheme. The feedback system control scheme consists of an iterative loop of three operations, including formulation of small molecule inhibitor combinations, experimental readouts of 'stemness', including number of alkaline phosphatase positive (AP+) colonies and percentage of OCT4-GFP expressing cells, and a search algorithm linking the cellular readouts and the cocktail combinations. On identification of small molecule cocktails capable of maintaining high OCT4 expression over a week, their ability in supporting long-term culture was tested through serial single cell passage up to 25 generations. Finally, the successful development of the small molecule-based defined culture condition was validated by the expression of various pluripotent markers, the capacity of teratoma formation and the maintenance of normal karyotype. Optimization strategy with feedback system control Our feedback system control scheme, as illustrated in Figure 1 , consists of an iterative loop of three operations, including formulation of small molecule inhibitor combinations, experimental readouts of 'stemness', and a search algorithm linking the cellular readouts and the cocktail combinations to generate new combinations for the subsequent rounds of experimental tests. Figure 1: A schematic illustration of our experimental design. Through literature search, five small molecule inhibitors targeting key pathways involved in hES cells were selected. Combinations and concentrations of the five inhibitors were optimized using the feedback system control scheme. The feedback system control scheme consists of an iterative loop of three operations, including formulation of small molecule inhibitor combinations, experimental readouts of 'stemness', including number of alkaline phosphatase positive (AP + ) colonies and percentage of OCT4-GFP expressing cells, and a search algorithm linking the cellular readouts and the cocktail combinations. On identification of small molecule cocktails capable of maintaining high OCT4 expression over a week, their ability in supporting long-term culture was tested through serial single cell passage up to 25 generations. Finally, the successful development of the small molecule-based defined culture condition was validated by the expression of various pluripotent markers, the capacity of teratoma formation and the maintenance of normal karyotype. Full size image We first defined a pool of small molecule inhibitors used in this study through a literature search, which led to five commercially available small molecule inhibitors that specifically target pathways associated with the differentiation, survival and proliferation of hES cells [3] , [27] , [28] , [29] , including mitogen-activated protein kinase (MEK) inhibitors PD98059 and PD0325901, a glycogen synthase kinase inhibitor (GSKi) CHIR99021, a Rho kinase inhibitor (ROCKi) Y27632 and a FGF receptor tyrosine kinase inhibitor (FGFRi) PD173074 ( Fig. 1 ). In addition, as hES cell maintenance likely depends on a very delicate balance of multiple signalling pathways, not only the specific combinations of the five small molecules but also their specific concentrations could be critical for the desired output. Therefore, six concentration levels that cover a 100-fold concentration range are considered for each inhibitor. These six concentrations are coded by numbers '0' to '5', where '0' has no inhibitor, whereas '3' being the concentrations found in the literature. Concentration '3' further serves as the 'base' for determining '1', '2' and '4', '5', concentrations either lower or higher from the base, respectively ( Table 1 ). Table 1 Concentrations and position sequence of the five small molecules used in the feedback system control. Full size table The success of the feedback system control heavily relies on the readouts that closely mimic the desired biological activity and the proper controls to evaluate the effects of the given small molecule combinations. As our goal is to maintain the 'stemness' of hES cells and promote cell proliferation, we decided to use number of alkaline phosphatase positive (AP + ) colonies as an initial readout because all measurement can be easily carried out on multi-well plates. However, AP + cells may not necessarily carry all properties of hES cells and may divert our selection process. Therefore, we genetically knocked the OCT4-GFP reporter construct into the endogenous OCT4 locus ( OCT4-GFP cells) of H1 and HSF1 hES cells [30] and used OCT4-GFP expression as the secondary confirmation readout. As a positive control, we used a current 'gold standard (GS)' of hES cell culture for single cell passaging, in which completely dissociated hES cells were plated on MEF cell-coated plates and cultured in hES cell medium supplemented with ROCK inhibitor Y27632 (ref. 3 ). In addition to the input and the readout, the search algorithm has an important role in efficiently guiding an exploration in such a large parameter space towards optimal combinations. Differential evolution (DE) algorithm, one of the well-established search game methods that mathematically exemplify a parallel search technique [31] , was chosen based on our successful application in identifying the optimal drug combination for reactivating virus [26] . The DE algorithm is briefly summarized in Supplementary Fig. S1 . The identified combinations/concentrations are then further tested on two independent hES cell lines, H1-OCT4-GFP and HSF1-OCT4-GFP, for their abilities to support the long-term (up to 25 serial passages) maintenance of hES cells through single cell passaging. Selection of defined surfaces and small molecule inhibitors To select a defined surface that would best support the culture of single hES cells and eliminate the need for feeder cells or Matrigel, we initially compared three defined surface conditions, including laminin, gelatin and polyethyleneimine (PEI), to conditions containing either MEF feeder cells or Matrigel at two different concentrations. These surface substrates were chosen based on their unique properties. For example, PEI is a synthetic polymer containing primary, secondary and tertiary amines, which provides a positively charged surface to attract negatively charged cell membrane to enhance surface attachment of ES cells [32] . In addition, laminin and gelatin have been shown to improve ES cell culture by providing extracellular matrix and structural scaffolding [16] , [33] , [34] , [35] . Interestingly, under the MEF-conditioned medium supplemented with ROCKi (CM+ Y27632), laminin supported more AP + colonies compared with PEI or gelatin and similar to Matrigel at 1:20 dilution ( Supplementary Fig. S2 ). As laminin is a major extracellular matrix protein component in Matrigel, we decided to use laminin as our first defined surface coating in subsequent studies. To determine whether the five small molecule inhibitors have collaborative effects on hES cells, we pre-tested their combinations at concentration levels of 0 and 3 (zero and base concentrations, Table 1 ) and analysed the number of AP + colonies after a 6-day culture period ( Fig. 2 ). To setup the experiments, hES cells were dissociated into single cells using accutase, and seeded onto various conditions at 2,500 cells per well in a 48-well plate. The positive control in this series of studies was the hES cell medium supplemented with 10 ng per ml bFGF, 20% knockout serum replacement (KSR) and Y27632 (ROCKi), deemed as the GS (red column). The negative control was hES cell medium without supplements or small molecules (open column or vertical arrow), whereas the testing conditions were negative control condition plus various combinations of small molecules. When cultured on MEF feeder cells, we saw a range of effects, from combinations outperforming the positive control (combinations left to the red column in Fig. 2a ), combinations falling in between the positive and the negative controls (between the red and open columns in Fig. 2a ) and combinations demonstrating inhibitory effects by producing fewer AP + colonies relative to the negative control (combinations right to the open column in Fig. 2a ). Overall, the top performers appeared to be combinations that consisted of either all or the majority of the inhibitors, whereas the inhibition was seen in combinations that consisted of simply GSKi, FGFRi or both ( Fig. 2a ). 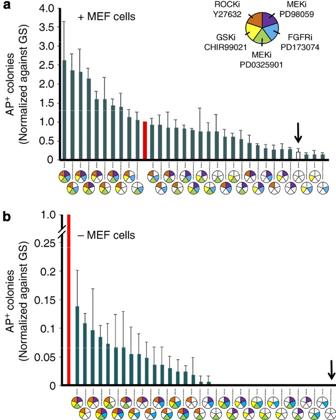Figure 2: Initial combinatorial trial of five small molecule inhibitors. Using two concentrations of each small molecule, corresponding to level '3' or '0' inTable 1, a total of 32 unique combinations were tested under two conditions: (a) MEF feeder cell-coated surface and (b) laminin-coated surface. The specific combinations are represented by the pie charts, in which positions and colours (filled or blank) of equally divided five sectors indicate inhibitors' identity and concentration ('3' or '0'), respectively. The number of AP+colonies in each combination was counted and normalized as fold of changes to the gold standard (GS, red columns). The open column and/or the solid arrow indicate the tested condition where no small molecules were added. The data are presented as the average of three independent tests (mean+s.d.). Figure 2: Initial combinatorial trial of five small molecule inhibitors. Using two concentrations of each small molecule, corresponding to level '3' or '0' in Table 1 , a total of 32 unique combinations were tested under two conditions: ( a ) MEF feeder cell-coated surface and ( b ) laminin-coated surface. The specific combinations are represented by the pie charts, in which positions and colours (filled or blank) of equally divided five sectors indicate inhibitors' identity and concentration ('3' or '0'), respectively. The number of AP + colonies in each combination was counted and normalized as fold of changes to the gold standard (GS, red columns). The open column and/or the solid arrow indicate the tested condition where no small molecules were added. The data are presented as the average of three independent tests (mean+s.d.). Full size image We next repeated the same study on a laminin-coated surface except for the positive control in which MEF feeder cells were present. The best combination supported roughly 15% as many AP + colonies as compared with the positive control (GS), suggesting a room for optimization using our feedback system control strategy ( Fig. 2b ). Interestingly, many of the top performers under the MEF feeder cell-containing conditions were the top performers under the laminin-coated conditions, indicating consensus among various combinations on the two surfaces. Defining optimal combinations via feedback system control With the demonstration that several combinations of the five small molecules may be able to support the culture of hES cells, we next attempted to improve the small molecule inhibitor cocktails by optimizing concentration of individual inhibitors using the feedback system control ( Fig. 1 ). For the first iteration, 32 initial combinations were randomly chosen using a random number generator in a numerical analysis software, MATLAB (Mathworks), and additional 32 trial combinations were generated by DE algorithm [31] using also a MATLAB program. For the subsequent iterations, 32 winner combinations from the immediately prior iteration and corresponding 32 trial combinations were tested. In each case, the GS was used as the positive control. During the initial iteration, the top performer of initial 32 random combinations delivered 37% as many AP + colonies as in the GS (black line in Fig. 3a ), whereas the best trial combination delivered 55% (purple line in Fig. 3a ). After the third iteration (blue line in Fig. 3a ), by which we cumulatively tested 128 out of 7,776 possible combinations, we obtained a condition (45030) that reached a similar number of AP + colonies as the GS ( Fig. 3a ), representing a roughly 2.5-fold improvement. Similar to our earlier studies shown in Figure 2a ranges of AP expression and cellular/colony morphologies were observed, suggesting a very unique cellular response per combination ( Supplementary Fig. S3a,b ). 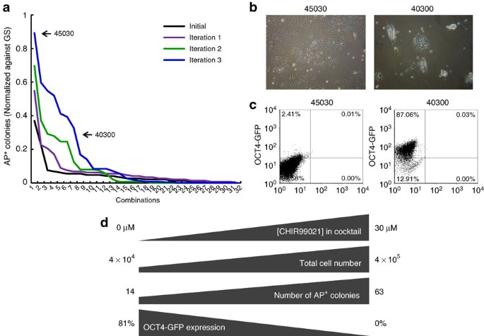Figure 3:APexpression-based iterations and the role of GSK inhibitor CHIR99021. (a) Increased AP+colony formation after each iteration step. The four data lines correspond to initial random combination, winners of the first iteration, second iteration and third iteration. Combinations 45030 and 40300 delivered 89.2 and 27.9% as many AP+colonies as the positive control, respectively. (b) Cellular morphologies of H1 cells cultured under combinations 45030 and 40300. (c)OCT4-GFPexpression of H1-OCT4-GFP cells cultured under combinations 45030 and 40300. (d) The effects of CHIR99021 concentration in hES cell culture. Although CHIR99021 supports the growth of hES cells and AP+colony formation, it also promotes their differentiation when used at higher concentrations, as indicated by the loss ofOCT4expression at 30 μM. Figure 3: AP expression-based iterations and the role of GSK inhibitor CHIR99021. ( a ) Increased AP + colony formation after each iteration step. The four data lines correspond to initial random combination, winners of the first iteration, second iteration and third iteration. Combinations 45030 and 40300 delivered 89.2 and 27.9% as many AP + colonies as the positive control, respectively. ( b ) Cellular morphologies of H1 cells cultured under combinations 45030 and 40300. ( c ) OCT4-GFP expression of H1-OCT4-GFP cells cultured under combinations 45030 and 40300. ( d ) The effects of CHIR99021 concentration in hES cell culture. Although CHIR99021 supports the growth of hES cells and AP + colony formation, it also promotes their differentiation when used at higher concentrations, as indicated by the loss of OCT4 expression at 30 μM. Full size image To determine whether AP staining could faithfully guide our search for 'stemness', we selected six combinations within the third iteration and repeated the studies on OCT4-GFP knock-in hES cell lines. Surprisingly, only one combination, 40300, delivered compact hES cell colonies and robust expression of OCT4-GFP ( Figs 3b,c and Supplementary Fig. S3c ). The most striking difference between 40300 and the other five conditions is the absence of the GSKi CHIR99021 (second position of the coding sequence; 0 versus 30 μM; Supplementary Fig. S3c ). To determine whether GSK inhibition is the determinant of such remarkable phenotype variations, we created a CHIR99021 gradient. As demonstrated in Figure 3d , CHIR99021 concentration positively correlates to the total cell number as well as AP + colonies, but negatively correlates to OCT4-GFP expression, with complete loss of OCT4-GFP at 30 μM CHIR99021 ( Supplementary Fig. S4 ). Although it is preferred to completely eliminate CHIR99021 from the combination mix and promote the undifferentiated status, 40300 produces tenfold less total number of hES cells as compared with 45030. Therefore, a balance of CHIR99021 will be necessary to attain a culture enabling system, which can enhance proliferation and achieve manufacturing scale production [36] . Refining culture systems for long-term hES cell maintenance With 40300 as candidate combination, we further refined our culture system by testing different basal media and extracellular proteins [7] , [8] , [17] , [20] for supporting OCT4-GFP hES cells. We compared both laminin and fibronectin alone or in combination in three different defined culture media, including DMEM/F12 supplemented with either 20% KSR, N2/B27 or simply insulin/transferrin/albumin (Minimal; Fig. 4a ). Compared with the GS (red column), every extracellular matrix protein(s) and medium combination supported hES cell growth, presented by both the percentage and total number of OCT4-GFP + cells, with fibronectin alone being the best ( Fig. 4a ). We therefore chose DMEM/F12 supplemented with 20% KSR and fibronectin surface combination for the next iteration series. Of note, while this manuscript was under review, four papers describing the use of synthetic surfaces [37] , [38] , [39] or laminin-511 (ref. 40 ) for long-term maintenance of hES cells were published. Although our study focuses on optimization of soluble small molecule inhibitors supporting maintenance of single-cell passaged hES cells, we also found that laminin and fibronectin to be the preferred surfaces for supporting hES cell maintenance, consistent with the recent publication [40] . 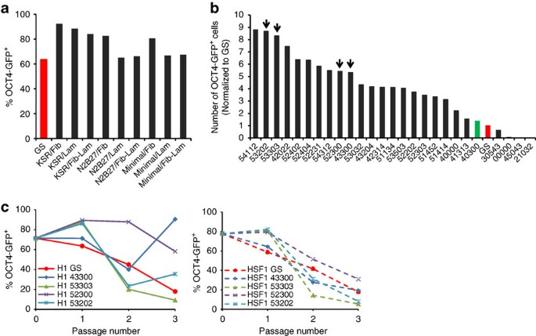Figure 4:OCT4-GFPexpression-based optimization. (a) Combination 40300 was tested in various media and on different extracellular matrix proteins. KSR, DMEM/F12 supplemented with 20% knockout serum replacement; N2B27, DMEM/F12 supplemented with N2 and B27 supplements; minimal, DMEM/F12 supplemented with transferrin, albumin and insulin. Results were presented as the percentage of OCT4-GFP+cells within the total number of viable cells. (b) After several OCT4-GFP-based iterations, top combinations (black arrows) were selected based on the total number of OCT4-GFP positive cells. Data are normalized to the gold standard (GS, red column) and can be directly compared with the starting combination 40300 (green column); 00000, no small molecules added. (c) Short-term passaging of H1-OCT4-GFP and HSF1-OCT4-GFP hES cells in GS and four selected combinations. All combinations, except for 43300 with H1-OCT4-GFP cells, failed to support high expressions ofOCT4-GFPover three continuous passages. Combination 43300, despite supporting a higher percentage of OCT4-GFP+cells, could not deliver a sufficient number of viable cells after three passages. Figure 4: OCT4-GFP expression-based optimization. ( a ) Combination 40300 was tested in various media and on different extracellular matrix proteins. KSR, DMEM/F12 supplemented with 20% knockout serum replacement; N2B27, DMEM/F12 supplemented with N2 and B27 supplements; minimal, DMEM/F12 supplemented with transferrin, albumin and insulin. Results were presented as the percentage of OCT4-GFP + cells within the total number of viable cells. ( b ) After several OCT4-GFP-based iterations, top combinations (black arrows) were selected based on the total number of OCT4-GFP positive cells. Data are normalized to the gold standard (GS, red column) and can be directly compared with the starting combination 40300 (green column); 00000, no small molecules added. ( c ) Short-term passaging of H1-OCT4-GFP and HSF1-OCT4-GFP hES cells in GS and four selected combinations. All combinations, except for 43300 with H1-OCT4-GFP cells, failed to support high expressions of OCT4-GFP over three continuous passages. Combination 43300, despite supporting a higher percentage of OCT4-GFP + cells, could not deliver a sufficient number of viable cells after three passages. Full size image As the scoring system based on AP + colonies rewarded cell proliferation rather than OCT4 expression, we then redefined our feedback loop by using OCT4-GFP expression as our new readout. After several iterations, we identified certain small molecule inhibitor combinations, which delivered more OCT4-GFP + cells as compared with the GS and 40300 combinations (red and green columns, respectively; Fig. 4b ). Although these combinations significantly outperformed the GS in terms of proliferation and the undifferentiated status, we needed bona fide proof that they can last the test of time during routine single cell passage. For this, two top combinations and two moderate combinations, along with the GS (indicated by arrows in Fig. 4b ) were tested for long-term assessments of hES cell maintenance. All combinations outperformed the GS at the first passage ( Fig. 4c , comparing red line with other lines). However, most combinations suffered a significant drop of OCT4-GFP expression during subsequent passages ( Fig. 4c ). Only combination 43300 was able to recover and maintain OCT4 expression at passage 3 ( Fig. 4c ). However, because of its low cell number, combination 43300 was also discontinued (data not shown). We reasoned that the drop of OCT4-GFP expression could be in part due to either the 'addictive' behaviour of hES cells to bFGF or passaging as single cell, as both H1 and HSF1 lines were generated and routinely cultured in the presence of bFGF [1] , [24] and have been passaged as clumps to maintain hES cell viability. To test the importance of bFGF, we repeated our long-term culture studies by adding 10 ng per ml bFGF to the 52300 combination (52300+bFGF), which performed better than the GS for both cell lines ( Fig. 4c ), and two other top combinations that significantly differed from 52300 (54112+bFGF and 42022+bFGF), along with 52300 and 43300 without bFGF ( Fig. 4b ). Remarkably, 52300+bFGF supported the maintenance of undifferentiated state of HSF1-OCT4-GFP and H1-OCT4-GFP cell lines for more than 25 serial passages without an adaptation period ( Fig. 5a ). This observation clearly supports the notion that hES cells are addictive to bFGF. However, as neither 00000+bFGF, 54112+bFGF or 42022+bFGF combinations can support OCT4 expression and/or cell growth, bFGF alone or together with other small molecule combinations is not sufficient for the maintenance of hES cells in long-term culture. These results highlight the uniqueness of combination 52300+bFGF in supporting hES cell maintenance. We also observed significant culture variations within H1-OCT4-GFP and HSF1-OCT4-GFP lines as HSF1-OCT4-GFP line adapted better to single cell passaging, even under 'non-bFGF' combination 43300, after an adjustment period ( Fig. 5a ). 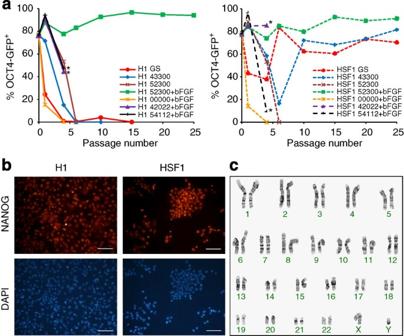Figure 5: Long-term single cell passaging and validation studies. (a) H1-OCT4-GFP and HSF1-OCT4-GFP lines were passaged in parallel in either GS or various small molecule combinations with or without bFGF for 25 passages (roughly 25 weeks), and the percentages of OCT4-GFP+cells were monitored periodically by fluorescence-activated cell sorting analysis. Black asterisks, cultures were terminated due to insufficient number of OCT4-GFP cells. (b) NANOG expression was analysed on H1-OCT4-GFP and HSF1-OCT4-GFP lines maintained in 52300+bFGF for 20 passages. Scale bars, 100 μm. (c) Normal karyotype of HSF1-OCT4-GFP cells was maintained after 21 continuous passages under 52300+bFGF. Figure 5: Long-term single cell passaging and validation studies. ( a ) H1-OCT4-GFP and HSF1-OCT4-GFP lines were passaged in parallel in either GS or various small molecule combinations with or without bFGF for 25 passages (roughly 25 weeks), and the percentages of OCT4-GFP + cells were monitored periodically by fluorescence-activated cell sorting analysis. Black asterisks, cultures were terminated due to insufficient number of OCT4-GFP cells. ( b ) NANOG expression was analysed on H1-OCT4-GFP and HSF1-OCT4-GFP lines maintained in 52300+bFGF for 20 passages. Scale bars, 100 μm. ( c ) Normal karyotype of HSF1-OCT4-GFP cells was maintained after 21 continuous passages under 52300+bFGF. Full size image Characterization of hES cells under the optimal condition To confirm the pluripotent status of hES cells beyond OCT4-GFP expression, we examined H1-OCT4-GFP and HSF1-OCT4-GFP cells cultured in parallel under GS and 52300+bFGF conditions for stage-specific embryonic antigen 4 (SSEA4) expression, NANOG expression, teratoma formation and genomic integrity during the course of 25 passages. Under 52300+bFGF, more than 90% of H1-OCT4-GFP and HSF1-OCT4-GFP cells remained positive for SSEA4 and NANOG ( Fig. 5b and Supplementary Fig. S5 ). HSF1-OCT4-GFP cells cultured in parallel under 52300+bFGF or the GS condition for 5, 15 and 20 passages were subcutaneously implanted into NOD/SCID/IL2γ null mice for teratoma formation. Histological analysis clearly indicated the development of heterogeneous tissues from the three embryonic germ layers ( Supplementary Fig. S6 ), demonstrating the ability of 52300+bFGF in maintaining the pluripotent state of hES cell during long-term culture. Furthermore, HSF1-OCT4-GFP cells cultured under 52300+bFGF successfully maintained normal karyotype ( Fig. 5c ) after 15 and 21 generations of continuous passaging, whereas cells in the parallel GS culture developed chromosome abnormalities ( Table 2 ) [41] . Although combination 43300 was able to support OCT4-GFP expression of HSF1-OCT4-GFP cells for 25 passages, we detected chromosome alterations after 15 generations of continuous passaging, suggesting that combination 43300 alone is not sufficient to maintain the genomic integrity of hES cells ( Table 2 ). Table 2 Karyotype of HSF1-OCT4-GFP cells. Full size table To demonstrate that our chemically defined culture conditions, including medium composition, substrate coating and seeding density, indeed support single cell culture, we conducted a clonal analysis by proportionally mixing GFP + HSF1-OCT4-GFP cells with GFP − parental HSF1 cells (GFP + :GFP − =0:100, 20:80, 40:60, 60:40, 80:20 and 100:0) and culturing/passaging under our standard seeding density on fibronectin-coated substrates. Six days post plating, GFP + , GFP − and mixed hES cell colonies were scored under the fluorescence microscope and quantified. As shown in Supplementary Fig. S7 , extremely low frequencies of mixed colonies (0–1.9%) were found within the range of dilutions, indicating that our defined culture condition is capable of supporting single cell culture. Taken together, our work demonstrates the uniqueness of three small molecule inhibitors against ROCK, GSK and MEK as well as bFGF in their defined concentrations (100 μM Y27632+0.95 μM CHIR99021+0.4 μM PD0325901+10 ng per ml bFGF) in supporting hES cell maintenance through single cell culture. In this study, we have demonstrated the ability of a unique set of small molecule inhibitors to support hES cell maintenance in a fully defined culture system. In addition, this culture system allows propagation of hES cells through a serial single cell passaging, which traditionally results in massive cell death. Our studies also suggest that bFGF has a key role in the maintenance of human ES cells through single cell passaging. Indeed, the addition of bFGF to combination of three small molecule inhibitors against ROCK, GSK and MEK delivered a culture system without a dramatic adaptation period and prevented loss of OCT4 expression. Derivation of new hES cells in media containing these three small molecule inhibitors without bFGF supplement will help decipher whether the dependence of bFGF observed in our study is due to the 'addictive' behaviour of H1 and HSF1 cell lines owed to their derivation and culture conditions or bFGF has a fundamental role in hES cell biology. It is also interesting to note that although high concentrations of GSK inhibitor, CHIR99021, promoted robust proliferation, it also facilitated the loss of OCT4 expression. Future studies may unveil the role of GSK inhibition on enhanced hES cell proliferation and differentiation for improving yields of specific cell types. The feedback system control methodology has proven to be invaluable in efficiently defining potent combinations of small molecule inhibitors for hES cell culture as previously demonstrated for viral infection inhibition and reactivation [25] , [26] . Successful identification of an enabling small molecule inhibitor cocktail required experimental testing of only 192 combinations out of 7,776 possible cases (128 cases for AP + colonies as readout and additional 64 cases for OCT4-GFP expression as readout). We have also realized that the output system is most critical to the success of this scheme. In our initial studies we used AP expression as our readout. Unfortunately, the expression of AP steered us towards cell number and away from undifferentiated state. On the other hand, the more stringent marker OCT4 allowed for an effective and faithful readout. We also observed significant variations among the two hES cell lines tested in this study. For example, although high CHIR99021 resulted in differentiation of both H1 and HSF1 cells, H1 cells are more sensitive to this inhibitor than HSF1 cells, a testament to the inherent difference observed among hES cell lines [42] . The current study represents a step forward in understanding the fundamental requirements of human pluripotent stem cell culture. It will be very interesting to unravel the specific biological effects that are elicited by combinations such as 52300 (short-term maintenance), 52300+bFGF (long-term maintenance) and 45043 (complete differentiation at passage 1). Taken together, our observations and finding suggest that similar to mouse ES cells [28] , the undifferentiated state of hES cells can be maintained in a fully defined culture system by a unique set of small molecule inhibitors through routine single cell passaging. Human embryonic stem cell culture Parental H1 and HSF1 lines as well as H1-OCT4-GFP and HSF1-OCT4-GFP lines were obtained from UCLA BSCRC Core Facility. Protocols for culturing hES cells were adapted and modified from WiCell Research Institute's published protocol ( http://www.wicell.org/index.php?option=com_content&task=category&sectionid=7&id=246&Itemid=248 ). In short, hES cells were routinely cultured in human ES cell medium containing DMEM/F12 (Invitrogen), 20% KSR (Invitrogen), 10 ng per ml bFGF (PeproTech), 1% Nonessential amino acids (Invitrogen), 2 mM L -Glutamine (Invitrogen), 0.1 mM 2-Mercaptoethanol (Sigma-Aldrich) on irradiated MEF cells in a 6-well tissue culture plate (BD Biosciences). Cells were passaged as clumps at a subculture ratio of 1:6 every 5–7 days using a dissociation solution consisting of Collagenase IV (1 mg ml −1 ; Sigma-Aldrich) and Dispase (1 mg ml −1 ; Sigma-Aldrich) in DMEM/F12. To initiate experiments with individually dissociated hES cells, at least 1 h before enzymatic cell dissociation, hES cell medium was replaced with hES cell medium supplemented with 10 μM Y27632 (Sigma-Aldrich or Ascent Scientific), a specific ROCK inhibitor [3] . Cells were then dissociated into single cells by incubating with pre-warmed Trypsin (Invitrogen) or Accutase (Invitrogen) for 5 min at room temperature, collected, pelleted by centrifugation (5 min at 200 g ), resuspended in the Y27632-supplemented hES cell medium, transferred to a gelatin-coated tissue culture plate and cultured for 1 h to remove MEF cells. hES cells that remained unattached were then collected and filtered through a 40 μm cell strainer (BD Biosciences) to remove cell aggregates. On counting number of viable cells using a Hemocytometer (Fisher Scientific), dissociated single cells were plated into tissue culture plates containing medium formulations to be tested. For subsequent passages, hES cells were enzymatically dissociated with accutase as described above, but without pre-incubation with the Y27632 supplemented medium and the MEF removal step. Preparation of surface coatings In preparation of various surfaces, Laminin (20 μg ml −1 ), Fibronectin (20 μg ml −1 ), Gelatin (2 mg ml −1 ), Polyethyleneimine (25 μg ml −1 ; all from Sigma-Aldrich), or Matrigel (1:20 and 1:200 dilutions: BD Biosciences) was used to coat each well of multi-well plates (300 μl for 48-well plates and 1 ml for 6-well plates) for 2–3 h and was aspirated immediately before introduction of hES cells. Preparation of small molecule cocktails Human ES cell wash medium (DMEM/F12+20% KSR+1% nonessential amino acids+2 mM L -glutamine+0.1 mM 2-mercaptoethanol) was used as a defined basal medium. The five inhibitors were first reconstituted into stock solutions; 1 mM Y27632 was prepared in DMEM/F12, and 10 mM CHIR99021, 4 mM PD0325901, 1 mM PD173074 and 50 mM PD98059 were prepared in dimethyl sulfoxide. Stock solutions were either stored at 4 °C (Y27632) or at −20 °C (the other four molecules) until use. Small molecule cocktails were prepared by adding corresponding amounts of the stock solutions to the filtered human ES cell wash medium ( Table 1 ). To avoid absorption of small molecules on the surface of plastic bottles due to hydrophobic interactions, sterile glass bottles were used to store formulated small molecule cocktails. Other basal medium formulations Throughout this paper the human ES cell wash medium was used as our choice of basal medium unless otherwise mentioned. Two other basal media were formulated and tested. DMEM/F12-N2B27 basal medium contains DMEM/F12, 1× N2 supplement, 1× B27 supplement, 1× L -glutamine, 1× nonessential amino acids, 0.1 mM 2-mercaptoethanol and 5 mg per ml BSA fraction V (all from Invitrogen). DMEM/F12 minimal basal medium contains DMEM/F12, 1× L -glutamine, 1× nonessential amino acids, 0.1 mM 2-mercaptoethanol and 5 mg per ml BSA fraction V, 10 μg per ml insulin, 10 μg per ml transferrin, and 0.1 μg per ml ascorbic acid (all from Invitrogen). Staining for alkaline phosphatase activity and NANOG For alkaline phosphatase activity analysis, hES cells cultured on multi-well plates were fixated with 10% formalin (Fisher Scientific), rinsed with PBS three times and stained using Vector Red Alkaline Phosphatase Substrate Kit I (SK-5100, Vector Laboratories). Images of stained wells were captured using CoolSNAP HQ CCD camera (Photometrics) mounted on Leica DM-IRB inverted fluorescent microscope (Leica Microsystems). For NANOG staining, hES cells were fixated with 10% formalin and permeabilized with 0.5% Triton-X (Sigma-Aldrich) in PBS for 10 min. After rinsing in 0.2% Tween 20 (Fisher Scientific) in PBS (wash buffer), the cells were blocked by incubating in 5% goat serum in PBS containing 0.2% Tween 20 (blocking buffer) for 15 min. After gently aspirating the blocking buffer, the cells were incubated overnight at 4 °C in the blocking buffer containing anti-NANOG antibody (1:500 dilution, Abcam). After rinsing three times with the wash buffer, the cells were stained using secondary antibodies conjugated to Alexa 546 or Alexa 488 (1:250 dilution, Invitrogen) in the blocking buffer and incubated for 1 h at room temperature. Following rinsing with the wash buffer and 4,6-diamidino-2-phenylindole staining, images of the stained wells were captured by using the inverted fluorescence microscope and the CCD camera. Flow cytometry analysis for OCT4-GFP and SSEA4 expressions For routine analysis of OCT4-GFP expression, cells were dissociated with accutase and centrifuged for 5 min at 200 g to remove cell debris. After removal of supernatant, cell pellets were resuspended in 300 ml of Hank's buffered salt solution (HBSS) containing 4% serum and kept on ice. For analysis of SSEA4 expression, pelleted cells by enzymatic dissociation and centrifugation as described above were resuspended in HBSS containing 4% serum and stained with Phycoerythrin (PE) anti-human SSEA4 antibody (1:100 dilution, eBioscience) for 15 min on ice, followed by centrifugation. The pelleted cells were then resuspended in HBSS containing 4% serum and kept on ice. For both samples, 7 μl of 7-Aminoactinomycin D (BD Biosciences) was added to stain non-viable cells ∼ 5 min before fluorescence-activated cell sorting analysis. The cell viability and OCT4-GFP and SSEA4 expressions were acquired and analysed with BD FACS Canto II Flow Cytometry System (BD Biosciences). Teratoma formation One million cells were mixed with Matrigel and implanted subcutaneously into the dorsal-flank region of NOD/SCID/IL2γ null mice. Four to six weeks post injection, teratomas were collected and analysed by hematoxylin and eosin staining to identify various cell types. Karyotype analysis Standard cytogenic analyses were performed on 20 G-banded metaphase cells by Cell Line Genetics. How to cite this article: Tsutsui, H. et al . An optimized small molecule inhibitor cocktail supports long-term maintenance of human embryonic stem cells. Nat. Commun. 2:167 doi: 10.1038/ncomms1165 (2011).